Microsphere-assisted fabrication of high aspect-ratio elastomeric micropillars and waveguides High aspect-ratio micropillars are in strong demand for microtechnology, but their realization remains a difficult challenge, especially when attempted with soft materials. Here we present a direct drawing-based technique for fabricating micropillars with poly(dimethylsiloxane). Despite the material’s extreme softness, our technique enables routine realization of micropillars exceeding 2,000 μm in height and 100 in aspect-ratio. It also supports in situ integration of microspheres at the tips of the micropillars. As a validation of the new structure’s utility, we configure it into airflow sensors, in which the micropillars and microspheres function as flexible upright waveguides and self-aligned reflectors, respectively. High-level bending of the micropillar under an airflow and its optical read-out enables mm s −1 scale-sensing resolution. This new scheme, which uniquely integrates high aspect-ratio elastomeric micropillars and microspheres self-aligned to them, could widen the scope of soft material-based microdevice technology. Micropillars made of poly(dimethylsiloxane) (PDMS) have seen rapid expansion in their application scope, from biomimetic dry adhesion [1] and surface wetting control [2] to cell mechanic studies [3] , [4] , [5] , [6] . That scope can be further widened by increasing their height and aspect-ratio. However, realizing PDMS micropillars with mm-scale heights, while keeping their diameters at μm-scale, remains a difficult challenge, especially when conventional, replica-molding-based fabrication techniques [7] were adopted. The main obstacle is the need to de-mold the PDMS micropillars after curing. Despite the efforts to improve the yield of the process [4] , [8] , the failure rate increases inevitably with the height and aspect-ratio. Another source of difficulty is the inherently low Young’s modulus of PDMS (typically ~1 MPa) [9] , which frequently leads to the collapse of the micropillars and their irreversible bonding to the substrate [10] . For these reasons, the height and aspect-ratio of PDMS micropillars have been capped at ~700 μm and ~20 μm so far, respectively [7] . Here we present a new technique that not only improves the achievable height and aspect-ratio of the PDMS micropillar but also enhances its functionality to a great extent. The key enabling factor is the adoption of the direct drawing technique. It exploits rapid solidification of the capillary bridge to eliminate the need for de-molding. To date, it has been applied to polystyrene [11] , PMMA [12] , PTT [13] , nylon [14] , sucrose [15] , polyurethane [16] , SU-8 (ref. 17 ) and adhesives [18] . Its application to PDMS, however, has not been reported due mainly to the material’s softness and slow solidification rate. We address the issues by incorporating in situ heating into the drawing process so that the micropillar gets simultaneously hardened and solidified during its formation. Such directly drawn PDMS micropillars can perform various functionalities, including the role of flexible upright waveguides thanks to the transparency of PDMS. A more interesting feature of our technique is the use of microspheres as the drawing probes, leading to the realization of microsphere-tipped micropillars (MSMPs). The microspheres can play multiple roles such as the enhancer of the micropillar’s tip-visibility [7] or the tip-mass, which tunes the micropillar’s motion dynamics. The fact that they are self-aligned to the micropillars further widens their application scope. To validate the utility of the PDMS MSMP, we configure it into airflow sensors. The micropillar functions as a vertical waveguide, which deforms under airflow, and the microsphere as a self-aligned reflector, which reports the micropillar’s level of deformation. Manual installation of such microspheres can be tedious and error-prone [7] . Our scheme, in contrast, integrates them in situ . Both the fabrication technique and the resulting structure, which uniquely combines high aspect-ratio micropillars and microspheres in a self-aligned manner, will open new possibilities in soft material-based microtechnology. Fabrication of microsphere-tipped PDMS micropillars We started out with the preparation of the drawing probe array ( Fig. 1a ). The microspheres were first assembled on a photolithographically patterned SU-8 grid and then transferred onto a piece of double-stick tape attached to a glass substrate. We used two types of microspheres as the drawing probes: ~50 μm-diameter PMMA microspheres and ~58 μm-diameter Ag-coated hollow glass microspheres. The latter was more effective for increasing the levels of reflection and tip-visibility. We then flipped the array and attached it to a micro-manipulator. We also spin-coated a thin (~25 μm) layer of PDMS and pre-baked it on a hot plate placed under the micro-manipulator ( Fig. 1b ). During the pre-bake, we lowered the microsphere array towards the PDMS thin film until the separation was reduced to 50 μm. Upon completion of the pre-bake, we further lowered the microsphere array so that it can physically contact and get immersed in the PDMS thin film ( Fig. 1c ). After 40 s of contact, we lifted the micro-manipulator at 144 μm s −1 , drawing PDMS micropillars ( Fig. 1d ). The temperature was maintained at 100 °C throughout these steps for simultaneous solidification and hardening of the PDMS micropillars. Completed micropillars were then post-baked at 100 °C for 2 h and at room-temperature for 24 h. Finally, we detached the double-stick tape from the MSMPs ( Fig. 1e ). For this, we first moved up the micro-manipulator holding the double-stick tape so that the MSMPs got elongated by 100%. The resulting tension induces gradual detachments of the microspheres from the tape. It could take several minutes. At this step, the main cause of failure is insufficient curing of the PDMS micropillar, which detaches the microsphere from the micropillar rather than from the tape. 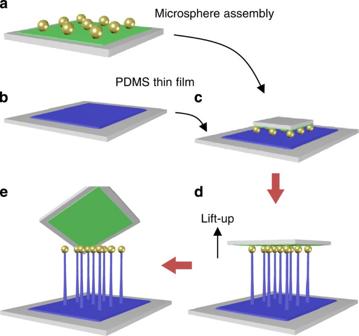Figure 1: Fabrication of microsphere-tipped PDMS micropillars. (a–e) Steps for direct drawing-based MSMP fabrication: (a) arraying of microsphere drawing probes on a piece of double-stick tape. (b) Spin-coating and pre-bake of a PDMS thin film. (c) Flip-contacting the microsphere array onto the PDMS thin film. (d) Micro-manipulator-assisted drawing of PDMS micropillars within situheating. (e) Removal of the double-stick tape upon the completion of the drawing process and post-bake. Figure 1: Fabrication of microsphere-tipped PDMS micropillars. ( a – e ) Steps for direct drawing-based MSMP fabrication: ( a ) arraying of microsphere drawing probes on a piece of double-stick tape. ( b ) Spin-coating and pre-bake of a PDMS thin film. ( c ) Flip-contacting the microsphere array onto the PDMS thin film. ( d ) Micro-manipulator-assisted drawing of PDMS micropillars with in situ heating. ( e ) Removal of the double-stick tape upon the completion of the drawing process and post-bake. Full size image Physical characteristics of PDMS micropillars The direct drawing technique enabled routine fabrications of mm-scale PDMS micropillars with aspect-ratios >40. Here, we defined the aspect-ratio as the ratio between h , the distance between the substrate and the micropillar-microsphere interface, and d ave , the average of the top, middle and base diameters. The micropillar in Fig. 2a was drawn with a 50 μm-diameter PMMA microsphere. With its h and d ave at 1,134 μm and 13.5 μm, respectively, the micropillar exhibits an aspect-ratio of 84. Such a high aspect-ratio was attainable for arrayed micropillars as well. The micropillars in the 4 × 4 array shown in Fig. 2b were drawn with a matching array of 58 μm-diameter Ag-coated hollow glass microspheres. In average, they were 877.2 μm high and tapered with their diameter changing from 14.4 μm right underneath the microsphere to 29.8 μm at the base. With 20.8 μm in d ave , their average aspect-ratio was 42. As pointed out above, capping the tip with a metallic microsphere greatly enhanced the micropillar’s tip-visibility. 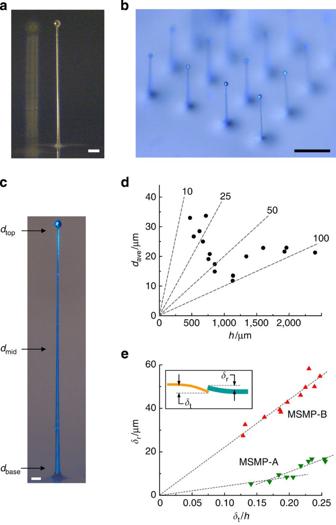Figure 2: Physical characteristics of the fabricated microsphere-tipped PDMS micropillars. Optical micrographs of (a) a 1,134 μm-high PDMS micropillar-integrated with a 50 μm PMMA microsphere. Its aspect-ratio is 84. (Scale bar, 100 μm), (b) a 4 × 4 array comprising 877.2 μm-high micropillars integrated with 58 μm Ag-coated hollow glass microspheres. (Scale bar, 700 μm), and (c) the micropillar with the highest aspect-ratio of 112 (dtop=9 μm,dmid=14 μm,dbase=41 μm andh=2.4 mm, scale bar, 100 μm). (d) The average diameterdaveof the micropillar plotted as a function ofh. The dotted lines mark the aspect-ratios. The data indicate that the aspect-ratio initially increases withhbut stabilizes in the range of 70~110 oncehexceeds ~1.1 mm. (e) The results of the reference-cantilever method-based measurements. The inset outlines the setup. The deflection length of the test cantilever (δt) induced by the reference cantilever with known mechanical properties was measured for different deflection levels (δr). The dotted lines represent the results of linear fit with zero or non-zerox-intersection assumed. Figure 2c shows the highest micropillar obtained so far. With its h and d ave at 2,400 μm and 21.3 μm, respectively, the aspect-ratio reached 112. To the best of our knowledge, this is the highest aspect-ratio reported for a vertical PDMS micropillar. Figure 2d shows the relation between h and d ave of our micropillars. Initially, the aspect-ratio increases with h . Beyond h ~1.1 mm, however, the increase in h induces a matching increase in the base diameter, saturating the aspect-ratio in the range of 70~110. Among the micropillars, we chose the three in Table 1 as our model components for further characterization and airflow-sensing application. Figure 2: Physical characteristics of the fabricated microsphere-tipped PDMS micropillars. Optical micrographs of ( a ) a 1,134 μm-high PDMS micropillar-integrated with a 50 μm PMMA microsphere. Its aspect-ratio is 84. (Scale bar, 100 μm), ( b ) a 4 × 4 array comprising 877.2 μm-high micropillars integrated with 58 μm Ag-coated hollow glass microspheres. (Scale bar, 700 μm), and ( c ) the micropillar with the highest aspect-ratio of 112 ( d top =9 μm, d mid =14 μm, d base =41 μm and h =2.4 mm, scale bar, 100 μm). ( d ) The average diameter d ave of the micropillar plotted as a function of h . The dotted lines mark the aspect-ratios. The data indicate that the aspect-ratio initially increases with h but stabilizes in the range of 70~110 once h exceeds ~1.1 mm. ( e ) The results of the reference-cantilever method-based measurements. The inset outlines the setup. The deflection length of the test cantilever ( δ t ) induced by the reference cantilever with known mechanical properties was measured for different deflection levels ( δ r ). The dotted lines represent the results of linear fit with zero or non-zero x -intersection assumed. Full size image Table 1 Characteristics of the PDMS micropillars under test. Full size table The simplicity of the MSMP fabrication process also renders it very robust. It took more than 140 pilot fabrications to optimize the process parameters such as the initial PDMS layer thickness, in situ curing temperature and drawing speed. Once they were optimized, we have experienced few failures when fabricating MSMPs one by one. Most failures occurred during the fabrication of MSMPs in an arrayed format. In both cases, the MSMP’s height and diameter exhibited finite spreads. The height of the MSMP could be controlled with μm-scale accuracy with the help of the micro-manipulator. The diameter, however, exhibited much wider spread. Our analysis revealed that both the spread in the diameter and the higher failure rate during arrayed fabrication arise from a common cause: the uncertainty in the depth of the microsphere’s immersion into the semi-cured PDMS film right before the drawing ( Fig. 1c ). Shallower (deeper) immersion inevitably decreases (increases) the contact area between the microsphere and the PDMS film, leading to thinner (thicker) MSMPs. Insufficient diameter leads to collapse of the micropillar. In contrast, micropillars that are too thick are more likely to fail during the detachment from the tape, which requires ~100% elongation. The immersion depth depends on a number of factors including the degree of PDMS curing, the size of the microsphere and the micro-manipulator’s contact force. In the case of arrayed fabrication, the tilting of the microsphere assembly is added as the dominant factor. The impacts of the immersion depth and contact area on the MSMP’s diameter accuracy and failure rate were clarified through the study of the 4 × 4 MSMP array in Fig. 2b . Among the 16 MSMPs, one failed due to excessive thickness during the detachment step. The s.d. in the height was only 10.35 μm for an average height of 877.2 μm. In contrast, the s.d. in the diameter was much greater: 5.25 μm for an average diameter of 20.8 μm. Supplementary Tables 1–3 show the maps of the MSMPs’ height, diameter and the diameter of the microsphere, respectively. The height map clearly shows that the microsphere array/double-stick tape composite ( Fig. 1c ) was slightly tilted, mainly along the direction of the table’s row, causing ~±15 μm deviations in the vertical positions of the microspheres and, hence, their immersion depths. The corresponding change in the MSMP’s diameter can be found in Supplementary Table 2 . 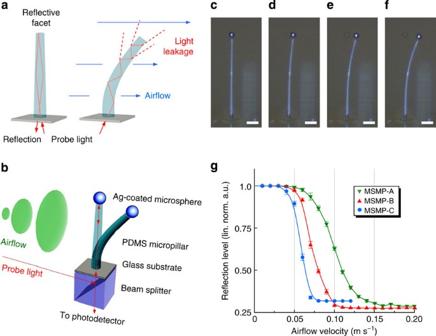Figure 3: Airflow sensing with microsphere-tipped high aspect-ratio PDMS micropillars. (a) The operation principle of the micropillar-based, optical airflow sensing. In the absence of an airflow, the micropillar stands upright, maximally reflecting the probe light. Under airflows, the micropillar bends, resulting in a reduction in the reflection level. (b) The optical read-out setup for MSMP-based airflow sensing. The three micropillars inTable 1were utilized. The surface of the Ag-coated microsphere functions as the reflective top facet of (a). Micrographs in (c–f) show the gradual increase in MSMP-A’s bending as the airflow velocity increases from 0 m s−1to 0.12 m s−1, 0.16 m s−1and 0.20 m s−1, respectively. (Scale bar, 100 μm) (g) The change in the micropillar’s reflection level as a function of the airflow velocity. The error bars represent the corresponding s.d. The commercial Ag-coated hollow glass microspheres we employed for this work came with a 53~63 μm diameter range and the measured diameters are listed in Supplementary Table 3 . Its correlation with the MSMP diameter is weaker than that of tilting. The fact that the only failure occurred to the corner MSMP, which suffers maximally from the tilt in both row and column directions, re-assures the importance of leveling the microsphere array before drawing. The minimum possible distance between two neighboring MSMPs, which in turn determines the attainable array density, is mainly limited by the following two factors. First, two neighboring micropillars tend to merge during the drawing process. At the early stage of drawing, significant axiconic pedestals are formed around the micropillars. They gradually diminish along the progress of drawing, but residual pedestals can still be observed around some MSMPs, as in Fig. 2c . When two micropillars under drawing were within the pedestal radius of each other, they would merge at a high probability. For micropillars drawn with the Ag-coated hollow glass microsphere (53~63 μm in diameter), the pedestal radius was 136.7 μm with 6.4 μm s.d. In practice, we experience few failures when drawing micropillars with their distance much greater than the pedestal radius ( Supplementary Fig. 1a ). Micropillar pairs with their distance shorter than or close to the pedestal radius, however, ended up in high rate of failure ( Supplementary Fig. 1b,c ). The second factor limiting the minimum possible distance is their elastic recoiling at the moment the microspheres got detached from the tape. As described in Results, the micropillars become elongated by almost 100% before freeing themselves from the tape. Their probability of hitting a neighboring one increases rapidly with their proximity. The optical loss of the MSMP is also important for their future utilizations as flexible optical waveguides. Optical loss of various waveguide materials, both organic and inorganic, and the corresponding waveguide propagation loss have been intensely investigated so far [19] , [20] . With ~20 μm in diameter and air-cladding, the MSMPs can support a large number of higher-order modes, making the surface roughness, rather than the material absorption, the main source of optical loss. It is difficult to directly measure the propagation loss of optical waveguides <3 mm in length. Previously, however, we have characterized lost wax-molded PDMS optical waveguides with cm-scale lengths and 100~200 μm diameters [21] , [22] . The AFM-measured surface roughness was in the range of 3.2±0.8 nm, and the corresponding waveguide propagation loss was <~3.5 dB cm −1 . For our current MSMPs are fabricated with no physical contact with molding structures, it will be reasonable to assume equal or lower surface roughness and propagation loss, which will be acceptable for their mm-scale operation lengths. Impact of in situ thermal hardening From the observations that the directly drawn PDMS micropillars can stand upright and support the weight of microspheres despite their thinness and high aspect-ratio, we conjectured that the in situ heating has indeed hardened PDMS. We quantified its impact by measuring the micropillar’s Young’s modulus E Y . Among many available methods [23] , [24] , we adopted the reference-cantilever method, shown in the inset of Fig. 2e , in which a reference cantilever with known spring constant K r is used to deflect the test cantilever and its spring constant K t is estimated from the relation K t · δ t = K r · δ r where δ t and δ r represent the deflection lengths of the test and reference cantilevers, respectively. For conically tapered beams, K and E Y are related by K =3π· E Y · d max 4 · T /(64· h 3 ) where T is the taper constant defined as d min / d max [25] . The three MSMPs in Table 1 were targeted for this characterization. The thin and long geometry of the PDMS micropillars and their material characteristics, which remains soft in absolute sense even after the thermal hardening, made it difficult to find adequate reference cantilevers. In our work, we chose a section of commercial PMMA fibre as the reference cantilever. Because the reported E Y of PMMA varied widely, we determined the E Y of our PMMA fibre by applying the reference-cantilever method to it with a section of communication-grade optical fibre as the reference cantilever. Since the optical fibre is made of high purity fused silica, we could use the tabulated E Y of fused silica to calculate K r , K t and eventually the E Y of the PMMA fibre. From the data in Supplementary Fig. 2 , it was estimated to be 3.0±0.18 GPa, which is close to the previously reported value (2.8 GPa), for a PMMA fibre from the same manufacturer [26] . We then applied the same method to the MSMPs using the PMMA fibre as the reference cantilever. For the first two MSMPs in Table 1 (that is, A and B), we could perform stable and consistent measurements of δ r and δ t while maintaining the δ t values below 25% of the MSMP height which, according to the rigorous large deflection beam theory [27] , [28] , leads to a linear relation between the applied force and the cantilever deflection. MSMP-C, the longest one, however, was too flexible to be kept within the regime of δ t / h <0.25 and excluded from the characterization. The measured δ r − δ t combinations are shown in Fig. 2e . In the case of MSMP-A, the δ r − δ t curve became nonlinear once δ r exceeded 150 μm, even though it is only ~20% of h , well within the linear regime. The corresponding increase in the δ r / δ t slope and E Y may be the outcome of strain hardening which, according to a recent study, becomes severer with decreasing structure dimensions [29] . So, we extracted the δ r / δ t slope only from the linear, small-deflection regime and estimated E Y based on it. For MSMP-A, the slope was ~0.0526. With d ave and h of the un-tapered reference cantilever at 21 and 2,600 μm, respectively, and those for the tapered ( T =0.45) MSMP-A at 19.8 and 800 μm, respectively, the estimated E Y of MSMP-A was approximately 2.45 MPa, which is higher than most E Y values reported for bulk PDMS (~1 MPa) [9] . Obtaining such a high E Y value in bulk PDMS requires hours of high temperature curing [30] . Beyond the point, the slope jumped to ~0.1414, suggesting even higher E Y . In the case of MSMP-B, we had to use an even thinner and longer PMMA fibre section ( d =15.4 μm, h =3517 μm) as the reference cantilever. The resultant δ t / δ r slope, shown in Fig. 2e , was constant around ~0.138. The corresponding E Y was ~2.31 MPa, which is very close to the MSMP-A estimate and still higher than typical bulk E Y values. We attribute the ~1 MPa increase in E Y to the in situ thermal hardening incorporated into the direct drawing process. Airflow sensing with microsphere-tipped micropillars To validate the utility of the PDMS MSMP, we turn it into optical airflow sensor for which both the high aspect-ratio and the microsphere-tipped architecture play essential roles. The outstanding flexibility of the material and the μm-scale diameter allow substantial flow-induced bending even in very short micropillars that can barely stand out above the stagnant boundary layer. A full exploitation of the merit, however, requires an effective read-out scheme that can accurately report the micropillar’s bending level. In our scheme, the microspheres play the enabling role as outlined in Fig. 3a,b . There, the PDMS micropillar functions as a flexible waveguide. The probe light enters the micropillar from the base and then gets reflected at the top facet back into the photodetector. The flow-induced bending of the micropillar reduces the reflection power through spoiled waveguiding and beam deflection. Critical to the success of the scheme is guaranteeing high-level reflection at the micropillar’s top facet. We accomplish it by capping the micropillar with an Ag-coated microsphere and used its surface as the reflector. Unlike those in existing work [7] , our microspheres are in situ installed in a self-aligned manner. Figure 3: Airflow sensing with microsphere-tipped high aspect-ratio PDMS micropillars. ( a ) The operation principle of the micropillar-based, optical airflow sensing. In the absence of an airflow, the micropillar stands upright, maximally reflecting the probe light. Under airflows, the micropillar bends, resulting in a reduction in the reflection level. ( b ) The optical read-out setup for MSMP-based airflow sensing. The three micropillars in Table 1 were utilized. The surface of the Ag-coated microsphere functions as the reflective top facet of ( a ). Micrographs in ( c – f ) show the gradual increase in MSMP-A’s bending as the airflow velocity increases from 0 m s −1 to 0.12 m s −1 , 0.16 m s −1 and 0.20 m s −1 , respectively. (Scale bar, 100 μm) ( g ) The change in the micropillar’s reflection level as a function of the airflow velocity. The error bars represent the corresponding s.d. Full size image We transformed the MSMPs in Table 1 into airflow sensors by adding the optical read-out setup shown in Fig. 3b . Figure 3c–f shows MSMP-A’s deformation in response to airflows with their velocities at 0 m s −1 , 0.12 m s −1 , 0.16 m s −1 and 0.2 m s −1 , respectively. In the absence of an airflow, as shown in Fig. 3c , the micropillar stands straight, producing maximal reflection. Upon contact with an airflow, it bends due to the fluidic drag force, resulting in a decrease in its reflection level. From numerical simulations described in Supplementary Note 1 , we found that the decrease can be ascribed to two mechanisms, that is, the spoiling of waveguiding and the deflection of the reflected light. The corresponding changes in the reflection levels are plotted in Fig. 3g for all three MSMPs. They commonly exhibit a quasi-linear regime sandwiched between two slowly varying curved regimes. The onset of the first curved regime can be defined as the threshold velocity of the MSMP-based airflow sensors. Figure 3g indicates that they were 0.07 m s −1 , 0.05 m s −1 and 0.04 m s −1 for MSMP A, B and C, respectively. The curves also indicate that the decrease in the reflection saturates beyond a certain velocity, forming a flat pedestal at 26~32% level. It is mainly due to the residual reflection at the air–glass interface, which is not affected by the airflow, and can be reduced with an antireflection coating. In the quasi-linear regime, the optically retrieved reflection level can function as a good measure of the airflow velocity. The data represent 10-measurement averages. For all three micropillars, the fluctuation in the measured reflection level was maximal near the midpoints of the quasi-linear regimes with the s.d. at 0.0215, 0.0208 and 0.0152 for MSMP A, B and C, respectively. The error bars represent the s.d. that is 0.2~3.8% of the mean values (1.67% in average). The slopes of the quasi-linear responses were −11.3 s m −1 , −17.8 s m −1 and −27.7 s m −1 for MSMP A, B and C, respectively. In conjunction with the s.d. obtained above, these slopes set the limits of detection at 1.82 mm s −1 , 1.16 mm s −1 and 0.55 mm s −1 for MSMP A, B and C, respectively, for steady state, non-time-varying, airflows. Movie files demonstrating flow-induced MSMP deformation can be found in Supplementary Movies 1 and 2 . Sensing of time-varying airflows We also investigated the utility of the MSMP for sensing airflows with time-varying flow-rates and directions, that is, sound waves. The output of a speaker, driven by 60~200 Hz sinusoidal voltage waves, functioned as the excitation for the three MSMPs of Table 1 . 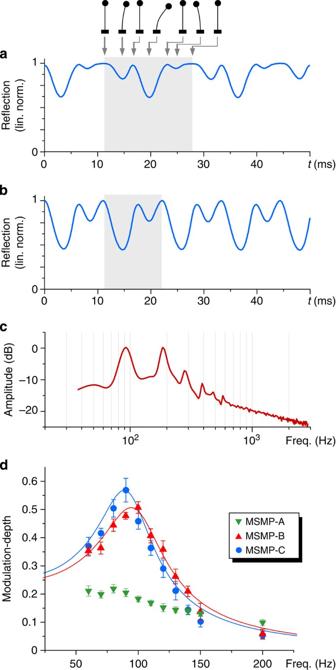Figure 4: Sound sensing with microsphere-tipped high aspect-ratio PDMS micropillars. (a,b) Temporally changing reflections from MSMP-C in response to sound waves at (a) 60 Hz and (b) 90 Hz. The shade indicates one temporal period. The inset in (a) is to explain the origin of the appearance of extra dips in the output. (c) The amplitude portion of the Fourier transform of the 90 Hz output. (d) The modulation-depth of the temporal responses from the three MSMPs ofTable 1as a function of the excitation frequency. The solid curves represent the results of fitting the data into the frequency response of the cantilever model described in Discussion. Error bars represent the s.d. obtained from five measurements. Figure 4a,b shows the optical reflection levels from MSMP-C responding to sound waves at 60 Hz and 90 Hz, respectively. The shades in the plots represent one temporal period. Given the sound wave driving the MSMP symmetrically, two identical dips per one temporal period were initially expected. The experimental results, however, exhibited severe asymmetry and, in the case of 60 Hz response, an extra dip. We attribute the asymmetry and the extra dip to the competition between the gradually increasing driving force and the restoration force of the PDMS micropillar. In the case of 60 Hz driving frequency, as shown in the inset of Fig. 4a , the MSMP had enough time to restore its original shape before the driving force finally reached its maximum, pushing it back into the maximal bending. As the driving frequency increases, the extra dip diminished and disappeared eventually ( Fig. 4b ). The resulting generation of higher harmonics is evident in the Fourier transform of the 90 Hz response ( Fig. 4c ). It indicates that the reflection waveform can provide accurate information on the frequency of the acoustic excitation, although it does not follow the exact excitation pattern. MSMPs A and B generated similar reflection patterns. Figure 4: Sound sensing with microsphere-tipped high aspect-ratio PDMS micropillars. ( a , b ) Temporally changing reflections from MSMP-C in response to sound waves at ( a ) 60 Hz and ( b ) 90 Hz. The shade indicates one temporal period. The inset in ( a ) is to explain the origin of the appearance of extra dips in the output. ( c ) The amplitude portion of the Fourier transform of the 90 Hz output. ( d ) The modulation-depth of the temporal responses from the three MSMPs of Table 1 as a function of the excitation frequency. The solid curves represent the results of fitting the data into the frequency response of the cantilever model described in Discussion. Error bars represent the s.d. obtained from five measurements. Full size image Figure 4d shows how the modulation-depth of the reflection output changes as a function of the excitation frequency over 60~200 Hz range. We tried our best to equalize the sound pressure at each frequency using a sound meter so that we can attribute the difference to the frequency dependence in the MSMP’s level of bending. The peak frequency f o could be easily identified for MSMP B and C as 102 Hz and 93 Hz, respectively. The response from MSMP-A, however, did not exhibit a definite peak within the test frequency range. Since the distance between our sound source and the MSMP was much shorter than the wavelength of the sound wave, the actual patterns of airflow around the MSMP could be much more complex than those of simple, sinusoidal waves. The analysis above may hold only at qualitative levels. Reports of theoretical framework for analyzing flexible micropillars with very high aspect-ratios, exceeding 40 as in the present work, are scarce. Here, we explore the effectiveness of the extended Euler–Bernoulli cantilever model for the analysis of our MSMPs. Its governing equation models the motion of a uniform, homogeneous, single-clamped cantilever beam due to a massflow by taking the impacts of inertia, bending, drag and viscous damping into consideration. It has been adopted by a number of researchers for flexible micropillars [31] , [32] , [33] . Traditionally, it has been used for absolutely linear bending for which the cantilever’s tip displacement d tip is below 5% of the cantilever length. The large deflection beam theory, which takes the bending into consideration as well, however, showed that the linear regime can be extended for the tip displacement up to 25% of the cantilever length [27] , [28] . Since the maximum tip displacement was less than 20% of the MSMP height in our experiments, we decided to try the linear model. The original equation depends on both the temporal and axial variations of the cantilever. We can assume a specific axial massflow pattern and integrate out the axial terms, resulting in an externally driven harmonic oscillator equation where m , c , k , F o and u ( t ) are to be determined from the structural and material characteristics of the cantilever, the magnitude and waveform of the driving force, and the axial profile of the massflow [33] . As described in Supplementary Note 2 , we utilized both linearly varying and constant axial massflow profiles [34] . The modelling results can be summarized as follows. First, with the structural, material and experimental parameters given above, the harmonic oscillator model of Eq. (1) could produce resonance frequency values that are in order-of-magnitude agreements with the experimental results. For example, the computed resonance frequencies for MSMP-B and C are in the range of 40~60 Hz, which is close to the measured values of 102 and 93 Hz. Second, by adjusting two material parameters, E Y and the density of PDMS ρ P , we could approximately reproduce the frequency responses of the two MSMPs. The results are superimposed in Fig. 4d . For MSMP-B, the best match was obtained with E Y =3.3 MPa and ρ P =525 kg m −3 , that is, half of the catalogue value. For MSMP-C, the best match required E Y =6.4 MPa and ρ P =525 kg m −3 . For MSMP-A, the shortest one, the predicted resonance frequency was 300~500 Hz. Since it was well beyond our experiment range, we did not try curve-fitting. Third, for both MSMP-B and C, better agreements were obtained when the massflow rate was assumed to be increasing linearly along the MSMP’s axis. Switching to the constant massflow profile lowered the resonance frequencies by a factor of 2 in both cases. The better match enabled by the adoption of the linearly varying flow-profile may indicate the persistent influence of the boundary layer even for cantilevers outstanding it by several hundred microns. These results indicate that application of the externally driven harmonic oscillator model to the highly flexible, high aspect-ratio PDMS micropillars could produce order-of-magnitude agreements in some output parameters. In general, however, the success was limited, necessitating more accurate numerical modeling. At this point, the MSMP-based airflow sensor’s performance should be assessed and compared with those of existing PDMS-based systems. There are two aspects: first, the MSMP’s effectiveness as an object interacting with an airflow. Second, the transduction mechanism that converts the changes in the MSMP into measurable signals. Regarding the first, the resonance frequency f o and the bandwidth constitute the main figures of merit. In this point of view, the significance of the MSMP comes from its height and the consequential red-shift in the f o . Replica-molded PDMS micropillars have been demonstrated by multiple researchers, but their height has been limited below 700 μm with the corresponding f o higher than 300 Hz, often in kHz range. For more versatile airflow sensing, lower frequencies need to be covered. The present MSMP, with the longest MSMP exhibiting f o near 100 Hz, has the potential to fill the gap. The microsphere-tipped nature of the MSMP may also enable further decrease in f o since the extra tip-mass can slow down the cantilever dynamics [35] . Currently, as shown in Fig. 4d , the overshoot near f o is less than 3 dB, which is reasonable for supporting wideband operation. In future designs, this flat, low-pass frequency response can be ensured through the control over the MSMP’s damping mechanisms. Regarding the transduction performance, the sensitivity would be the main figure of merit. Those for the MSMP-based sensors have already been evaluated in the previous section. Fair comparison with other cantilever beam-based airflow sensors [36] , however, is difficult since all of them utilized piezoelectric or capacitive read-out schemes. The only systems utilizing optical read-out were the PDMS micropillar wall shear-stress sensors relying on camera-based image capture and processing [7] , [32] . There, the sensitivity was defined as the ratio between the tip deflection amplitude and the wall shear stress and estimated to be ~150 μm Pa −1 for a 200 μm-high micropillar (20 in aspect-ratio) near 100 Hz. It was also predicted that the sensitivity would increase with the aspect-ratio in proportion to ( h / d ) 4.5 ~( h / d ) 5 . Figure 3d shows that the 1,600 μm-high MSMP-B (72.7 in aspect-ratio) exhibited deflection amplitude close to 20% of its height under 0.12 m s −1 airflow. Under the assumption of linearly increasing airflow velocity from the surface, the corresponding sensitivity is 0.25 m Pa −1 , which is in order-of-magnitude agreement with the sensitivity of the existing PDMS micropillar multiplied by (72.7/20) 5 . To summarize, the present MSMPs exhibit sensitivity comparable to existing PDMS micropillars while bringing in additional advantages of higher aspect-ratios and lower resonance frequencies. These sensitivity levels may be lower than those attainable with piezoelectric or capacitive read-out. Here we emphasize the optical read-out scheme’s unique advantages such as structural simplicity, spark-free operation and immunity to electromagnetic interference. The present scheme also exhibit advantages over existing optical read-out schemes, which rely on camera-based image capture and processing [7] , [32] , on the basis of its integration potential. For practical use, the reflection power measurement setup in Fig. 3b can be miniaturized and wafer-level integrated with CCD or CMOS detector arrays in an alignment-free manner [37] using beam redirection technologies developed for board-level optical interconnect. Integrating MSMPs with diverse characteristics will also allow simultaneous sensing of multiple frequency excitations. Currently, the biggest concern is the rather high measurement threshold, evident in Fig. 3g . Further modifications in the read-out configuration are required to address the issue. In conclusion, we report the development of a new softlithography technique with which we can draw high aspect-ratio PDMS micropillars. Despite the material’s inherent softness, the technique enables routine realization of vertical PDMS micropillars that measure 800~2,400 μm in height but only 25 μm or below in diameter. The resulting aspect-ratios, ranging from 40 to 112, are unprecedented for PDMS structures standing upright on their own. A more significant feature of our new fabrication technique is its ability to integrate microspheres at the tips of the micropillars in a self-aligned manner. To validate the utility of the microsphere-tipped PDMS micropillar, we turned it into a new type of airflow sensor in which the micropillar functions as a flexible optical waveguide. The self-aligned microspheres provide robust, high-level reflection to the waveguided probe light, enabling all-optical read-out of the micropillar’s deformation level. The high aspect-ratio and the excellent flexibility of PDMS synergistically enhance the micropillars’ level of deformation under airflows, leading to mm s −1 -scale resolution in airflow velocity sensing. The increase in the micropillar height also lowers their resonance frequencies from kHz range down to ~100 Hz, filling the gap in the operation bandwidth of microscale airflow sensing. The scope of application for the self-aligned microspheres can be further expanded with judicious choices on the microspheres’ size and composition. Overall, our new technique to realize microsphere-tipped high aspect-ratio micropillars will constitute a useful addition to the arsenal of soft material-based microtechnology. Drawing probe preparation Ag-coated hollow glass microspheres with 53~63 μm in diameter (M-40, Cospheric, 0.49 g cc −1 ) and PMMA microspheres with 45~53 μm in diameter (PMPMS-1.2, Cospheric, 1.2 g cc −1 ) were utilized to draw micropillars from PDMS (Sylgard 184, Dow Corning). To fabricate regularly arrayed micropillars, we first loaded the microspheres into an array of 30 μm-deep, 100 μm-diameter pits made of SU-8 2075 (MicroChem) through photolithography. Subsequently, we transferred the array onto a piece of double-stick tape (3 M) attached to a glass substrate. Then, we flipped the array and attached it to a micro-manipulator (MP-285, Sutter Instrument). Micropillar drawing A 10:1 wt ratio mixture of PDMS and its curing agent was spin-coated onto a glass slide (25 × 75 × 1.0 mm 3 , Fisherbrand) for 10 s at 500 r.p.m., then 45 s at 3,500 r.p.m., leading to a 25 μm-thick PDMS thin film. Then the PDMS thin film was placed on a 100 °C hot plate under the micro-manipulator and pre-baked for 140 s. During the pre-bake, we lowered the microsphere array towards the PDMS thin film until they got separated by 50 μm. Upon completion of the pre-bake, we further lowered the microsphere array to make it physically contact the PDMS thin film. After 40 s of contact, we lifted the micro-manipulator at a speed of 144 μm s −1 to directly draw PDMS micropillars. To solidify the micropillars formed between the microsphere array and the PDMS thin film completely, we post-baked it for 2 h at 100 °C and for 24 h at room temperature. Then, we manually detached the double-stick tape from the microspheres, completing the realization of the microsphere-micropillar complex. Young’s modulus measurement We measured the Young’s modulus of the PDMS micropillar through the length of its deflection induced by a PMMA fibre (MF0100, 100 μm in diameter, Paradigm Optics). The Young’s modulus of the PMMA fibre itself was measured with a section of communication-grade-fused silica optical fibre (Corning, SMF-28) as the reference. To facilitate the measurement, we thinned down the diameter of the PMMA fibre, which generally exhibits higher Young’s modulus than that of PDMS, to 20 μm through 330 s acetone bath. For the characterization of MSMP-B, we thinned it further down to 15.4 μm. Then, we pressed the thinned PMMA fibre on the test PDMS micropillar using a linear translation stage (9064-XYZ, Newport). The deflection lengths of the PMMA fibre and the PDMS micropillar were measured under a microscope (E-Zoom6, Edmund Optics). Airflow and sound sensing The characterization setup to verify the feasibility of MSMP-based airflow sensing is depicted in Fig. 3b . The probe light from a HeNe laser (632.8 nm, 0.95 mW, Thorlabs) is coupled into the flexible waveguide through a convex lens and a beam splitter so that it hits the microsphere at the tip of the flexible waveguide and then gets reflected back to be detected by the photodetector (918D-SL, Newport). For the best performance, the beam must hit the PDMS waveguide with a high degree of concentricity and parallelism. With the base diameter d base ranging from 30 to 43 μm, centering the weakly focused beam, diameter of which comparable to d base , to the base was straightforward with the help of a 3-axis linear stage equipped with three micrometers. The parallelism was achieved with the help of a separate tilt stage holding the MSMP/glass slide complex. These alignment steps were cumbersome but manageable with the help of the linear and tilt stages. The reflection data were acquired by a data acquisition board (NI 9215, National Instruments). Throughout our experiments, we set the sampling rate at 10 4 s −1 . A home-made LABVIEW program was used for data processing. In addition, we utilized compressed dry air (CDA) as the source of uniform airflows. The CDA line length beyond the flow-controller was approximately 70 cm. The CDA flow rate was controlled by a flow-controller (FMA 5518, Omega) from 0.01 to 0.2 m s −1 . We used the flow-controller readings as the estimates for the flow-rate in recording the experimental results, even though there could be discrepancies due to various fluid-dynamic effects. The distance between the micropillar and the airflow nozzle was 1.5 cm. As the source of the sound airflows, which is time-varying air-flows, we used a speaker (NS-3006 subwoofer, Insignia) driven by sinusoidal voltage waves taken from the computer board. The distance between the micropillar and the speaker was 10 cm. In addition, sound pressure at each frequency was equalized to be 95 dB using a sound level meter (PSPL01, PYLE). How to cite this article: Paek, J. & Kim, J. Microsphere-assisted fabrication of high aspect-ratio elastomeric micropillars and waveguides. Nat. Commun. 5:3324 doi: 10.1038/ncomms4324 (2014).